The 40-residue insertion inVibrio choleraeFadR facilitates binding of an additional fatty acyl-CoA ligand FadR is a master regulator of fatty acid metabolism and influences virulence in certain members of Vibrionaceae. Among FadR homologues of the GntR family, the Vibrionaceae protein is unusual in that it contains a C-terminal 40-residue insertion. Here we report the structure of Vibrio cholerae FadR ( Vc FadR) alone, bound to DNA, and in the presence of a ligand, oleoyl-CoA. Whereas Escherichia coli FadR ( Ec FadR) contains only one acyl-CoA-binding site in each monomer, crystallographic and calorimetric data indicate that Vc FadR has two. One of the binding sites resembles that of Ec FadR, whereas the other, comprised residues from the insertion, has not previously been observed. Upon ligand binding, Vc FadR undergoes a dramatic conformational change that would more fully disrupt DNA binding than Ec FadR. These findings suggest that the ability to bind and respond to an additional ligand allows FadR from Vibrionaceae to function as a more efficient regulator. Fatty acids (FAs) are major components of cell membranes and play important roles in energy metabolism. FadR is a member of the GntR family of transcription factors that coordinately controls the pathways of FA degradation and unsaturated fatty acid (UFA) biosynthesis in enteric bacteria [1] . In the absence of exogenous long-chain fatty acids (LCFAs), FadR functions as a repressor of FA degradation by binding to a site in the promoters of the fad genes and interfering with RNA polymerase [2] ( Fig. 1a ). These genes include fadL , fadD , fadBA , fadE and fadH that encode proteins required for the transport, activation and β-oxidation of LCFAs [3] . In V. cholerae , FadR also represses the expression of the plsB gene involved in membrane phospholipid biosynthesis [4] . In the absence of exogenous LCFAs, FadR simultaneously activates the expression of the fabA and fabB genes that encode proteins required for the biosynthesis of UFAs [5] , [6] . When exogenous LCFAs are present ( Fig. 1b ), they are transported across the outer membrane by FadL and activated by the inner membrane-associated acyl-coenzyme A (CoA) ligase FadD [7] to produce long-chain fatty acyl-CoAs (LCFA-CoAs). These LCFA-CoAs bind directly to FadR and induce a conformational change that releases FadR from its binding sites [8] . This derepresses fad gene expression to utilize the LCFAs and decreases the expression of fabA and fabB since UFA biosynthesis is no longer necessary. 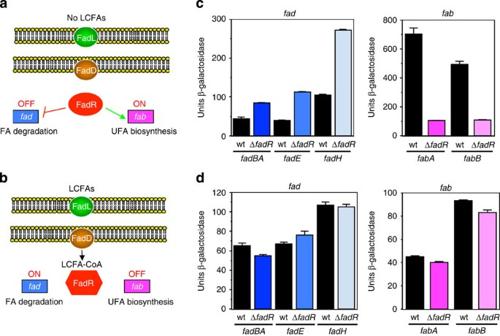Figure 1: Roles of FadR inV. cholerae. (a,b) Schematic showing FadR-mediated regulation inV. cholerae. In the absence of LCFAs, (a) FadR represses FA degradation by binding to a site in the promoters of thefadgenes and activates UFA biosynthesis by binding to a site in the promoters of thefabAandfabBgenes. In the presence of LCFAs, (b) they are transported into the cell by FadL and activated to LCFA-CoAs by FadD. The resulting activated LCFA-CoAs bind to FadR causing a conformational change that releases it from DNA and results in derepression and failure to activate its regulated promoters. (c,d) Influence of a ΔfadRmutation on the expression offadBA, fadE, fadH, fabA and fabBpromoter-lacZfusions inV. cholerae. Strains were grown in Tryptone medium with aeration for 5 h at 37 °C in the absence (c) and presence (d) of 2.5 mM oleate. From left to right: WL1031 (fadBA-lacZ), WL1035 (ΔfadR), WL1027 (fadE-lacZ), WL1029 (ΔfadR), WL1040 (fadH-lacZ), WL1042 (ΔfadR), WL1005 (fabA-lacZ), WL1007 (ΔfadR), GK1609 (fabB-lacZ) and GK1610 (ΔfadR). Error bars indicate the s.d. of at least two replicates. Results are representative of at least three independent experiments. Figure 1: Roles of FadR in V. cholerae. ( a , b ) Schematic showing FadR-mediated regulation in V. cholerae . In the absence of LCFAs, ( a ) FadR represses FA degradation by binding to a site in the promoters of the fad genes and activates UFA biosynthesis by binding to a site in the promoters of the fabA and fabB genes. In the presence of LCFAs, ( b ) they are transported into the cell by FadL and activated to LCFA-CoAs by FadD. The resulting activated LCFA-CoAs bind to FadR causing a conformational change that releases it from DNA and results in derepression and failure to activate its regulated promoters. ( c , d ) Influence of a Δ fadR mutation on the expression of fadBA, fadE, fadH, fabA and fabB promoter- lacZ fusions in V. cholerae . Strains were grown in Tryptone medium with aeration for 5 h at 37 °C in the absence ( c ) and presence ( d ) of 2.5 mM oleate. From left to right: WL1031 ( fadBA-lacZ ), WL1035 (Δ fadR ), WL1027 ( fadE-lacZ ), WL1029 (Δ fadR ), WL1040 ( fadH-lacZ ), WL1042 (Δ fadR ), WL1005 ( fabA-lacZ ), WL1007 (Δ fadR ), GK1609 ( fabB-lacZ ) and GK1610 (Δ fadR ). Error bars indicate the s.d. of at least two replicates. Results are representative of at least three independent experiments. Full size image In addition to controlling the activity of FadR, UFAs, which are components of bile in the intestinal lumen, are important signals present in the host environment that influence the expression of virulence genes in V. cholerae [9] . Members of Vibrionaceae are ubiquitous in marine and fresh water environments, with species found in open water, estuaries and marine sediments as either free-living or in association with phyto- and zooplankton [10] , [11] . V. cholerae is the causative agent of the acute intestinal infection cholera. Upon entry into the host intestine, V. cholerae induces a transcriptional cascade resulting in the expression of the AraC-type master virulence regulator, ToxT. ToxT directly activates the expression of the two primary virulence factors of V. cholerae , the toxin-coregulated pilus [12] and cholera toxin [13] . UFAs have been found to directly bind into the pocket of ToxT and influence its activity by impairing the ability of the protein to dimerize and bind to DNA [14] , [15] . The location of the UFA, buried in the ligand pocket at the interface between the N- and C-terminal domains is thought to promote a ‘closed’ conformation of ToxT that is not capable of binding to DNA. Once the bacteria have penetrated the mucus of the intestine, and the concentrations of UFAs are reduced, the closed conformation is presumably destabilized and the protein becomes competent for DNA binding and activation of gene expression [14] . The majority of FadR proteins that have been identified are members of the GntR family, as typified by E. coli FadR ( Ec FadR), which has been crystallized in its apo, ligand-bound and DNA-bound forms [16] , [17] , [18] . Ec FadR has an N-terminal DNA-binding domain containing a winged helix-turn-helix (wHTH) motif, and a C-terminal domain consisting of a seven-helical bundle containing a large cavity that is involved in acyl-CoA binding [16] . Upon ligand binding, effector-induced conformational changes occur in the protein that lead to displacement of the entire DNA-binding domain with respect to the effector-binding domain, leading to disruption of the protein–DNA complex [17] . FadR from Vibrionaceae is unusual among FadRs of the GntR family in that it contains a 40-amino-acid insertion in its C-terminal domain [19] . Although FadR from V. cholerae appears to repress gene expression as well as other FadR homologues that have been examined, it has a higher binding affinity for acyl-CoAs than the other homologues and it induces the expression of genes involved in FA utilization (that is, it is derepressed) more efficiently in the presence of ligand [19] . It has been suggested that these properties may be related to the 40-amino-acid insertion confined to the family. To gain insights into the role of this 40-amino-acid insertion for V. cholerae FadR ( Vc FadR), we have crystallized the Vc FadR protein in three forms: apo, bound to its cognate DNA and in the presence of a ligand, oleoyl-CoA. Our results indicate that the insertion region in Vc FadR potentially stabilizes the wing of the wHTH DNA-binding domain in the absence of DNA and, strikingly, facilitates the binding of a second oleoyl-CoA ligand in each monomer. The large conformational changes that occur in the protein upon binding of this second ligand are predicted to more fully disrupt DNA binding than what has been observed in the E. coli protein, possibly explaining why Vc FadR is a more efficient regulatory protein. Vc FadR is unusual but still regulates FA metabolism FadR is present in a variety of bacterial species where it plays a role in the transcriptional regulation of genes involved in FA metabolism [20] . The regulation of genes involved in FA degradation and UFA biosynthesis by FadR in V. cholerae has been inferred from bioinformatics analyses [20] , [21] . To confirm that Vc FadR functions as a regulator of these processes in V. cholerae , fusions of a promoterless lacZ gene from E. coli were made to the upstream regions of the V. cholerae fadBA , fadE and fadH genes involved in FA degradation and to the fabA and fabB genes involved in UFA biosynthesis. The fusions were introduced into the V. cholerae chromosome at the lacZ locus, and examined in the presence and absence of FadR and LCFAs. As shown in Fig. 1c , the loss of FadR increased the expression of the fadBA , fadE and fadH promoters 2-, 2.8- and 2.5-fold, respectively, whereas it decreased the expression of the fabA and fabB promoters 6.7- and 4.5-fold, respectively, in the absence of LCFAs. In the presence of LCFAs ( Fig. 1d ), no significant difference in the expression of the fusions was observed between the wild-type and Δ fadR mutant strains. These results show that FadR functions as a regulator of FA metabolism in V. cholerae . Vc FadR shares 52% sequence identity with Ec FadR ( Fig. 2a ). However, the protein from V. cholerae , as well as from other members of Vibrionaceae , shows a major difference from all other GntR family FadRs that have been sequenced in that it contains 40 additional residues in the C-terminal domain ( Fig. 2a,b and Supplementary Fig. 1 ). A Blast search [22] with V. cholerae FadR also reveals several related proteins with a 44-residue insertion ( Supplementary Fig. 1 ). Thus, it appears that Vibrionaceae FadRs acquired an insertion at some point in their evolution; retention of this insertion suggests that it provides a biological advantage for the organism. 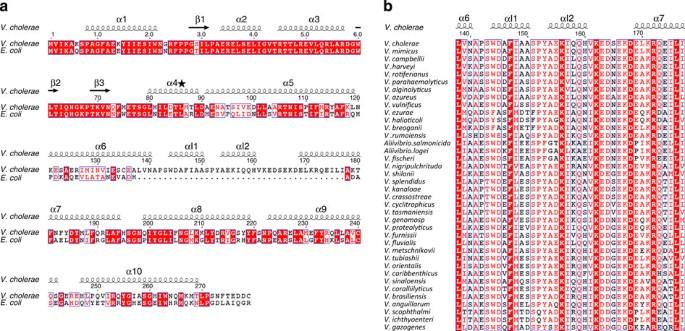Figure 2: Sequence alignment of FadR. (a) Alignment of FadR betweenV. choleraeandE. coli. Identical residues are indicated by red background. Incomplete identities among aligned sequences are in red text. Secondary structure is shown above the sequence and the numbering is based onEcFadR (PDB 1E2X)16. Helix α4, marked with the star, undergoes a helix-to-loop transition upon ligand binding. (b) Alignment of 40-residue insertions fromVibrionaceae. Colours are the same as ina. The alignments were prepared with Clustal W42and ESPript 3.0 (ref.43,http://espript.ibcp.fr/). Figure 2: Sequence alignment of FadR. ( a ) Alignment of FadR between V. cholerae and E. coli . Identical residues are indicated by red background. Incomplete identities among aligned sequences are in red text. Secondary structure is shown above the sequence and the numbering is based on Ec FadR (PDB 1E2X) [16] . Helix α4, marked with the star, undergoes a helix-to-loop transition upon ligand binding. ( b ) Alignment of 40-residue insertions from Vibrionaceae . Colours are the same as in a . The alignments were prepared with Clustal W [42] and ESPript 3.0 (ref. 43 , http://espript.ibcp.fr/ ). Full size image Structure of apo- Vc FadR and comparison with Ec FadR To shed light on the role of the insertion for Vibrionaceae , the structure of V. cholerae apo-FadR was determined ( Fig. 3a and Table 1 ). The asymmetric unit contains a dimer formed in a manner similar to that of Ec FadR (PDB 1E2X and 1HW1) [16] , [18] . Each monomer consists of an α/β N-terminal domain (residues 2–72, α1-β1-α2-α3-β2-W1-β3-W2, ‘W’ denotes a ‘wing’), a helical C-terminal domain (residues 94–279, α5−α6−αI1-αI2-α7-α8−α9−α10, ‘I’ denotes that the helix is derived from the insertion) and a short helical linker (residues 81–89, α4; Fig. 3a ). The structure of the N-terminal domain conforms to the so-called wHTH motif [23] , consistent with its role in binding DNA, and contains the most flexible loop in the structure as suggested by its B-factors ( Supplementary Fig. 2a ). 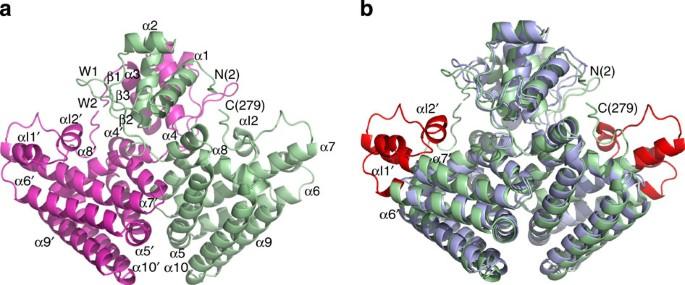Figure 3: Structure ofVcFadR. (a) TheVcFadR dimer. One monomer is magenta and the other is green. The N and C termini are labelled and the amino-acid positions are shown in parentheses. αI1 and αI2 denote the helices from the insertion and W1 and W2 denote wings. Helices from chain B are distinguished by a prime. (b) Superposition of the structures of theVcFadR andEcFadR dimers (PDB 1E2X). The 40-residue insertion inVcFadR is red and the rest of the protein is green.EcFadR is shown in blue. Figure 3: Structure of Vc FadR. ( a ) The Vc FadR dimer. One monomer is magenta and the other is green. The N and C termini are labelled and the amino-acid positions are shown in parentheses. αI1 and αI2 denote the helices from the insertion and W1 and W2 denote wings. Helices from chain B are distinguished by a prime. ( b ) Superposition of the structures of the Vc FadR and Ec FadR dimers (PDB 1E2X). The 40-residue insertion in Vc FadR is red and the rest of the protein is green. Ec FadR is shown in blue. Full size image Table 1 Data collection and refinement statistics. Full size table Superposition of the Vc FadR dimer on the Ec FadR dimer (PDB 1E2X) [16] ( Fig. 3b ) reveals that overall the two proteins are very similar (root mean square deviation over 424 alpha carbon atoms is 1.64 Å) except for the insertion (residues 138–177), which lies between helix α6 and helix α7. The insertion region elongates helices α6 and α7, as previously predicted [19] , and forms two additional short α-helices, αI1 and αI2, along with several connecting loops. Structure of Vc FadR with DNA and comparison with Ec FadR Vc FadR was crystallized in complex with a 31-bp oligonucleotide derived from the V. cholerae fadBA promoter ( Fig. 4a,b and Table 1 ). As in the Ec FadR–DNA complex (PDB 1H9T and 1HW2) [17] , [18] , the DNA-binding site is recognized by residues from helices α1, α2 and α3, which interact with the major groove, as well as the two wings (W1 and W2) that bind to the adjacent minor grooves ( Fig. 4a,c ), stabilizing these loops significantly ( Supplementary Fig. 2b ). As in the Ec FadR–DNA complex, the DNA in the V. cholerae FadR–DNA complex has a B-form conformation with a curvature of ~20° towards the protein, resulting in a contraction of the central major groove and an expansion of the opposite minor groove. As the amino-acid sequences of the DNA-binding domains of the V. cholerae and E. coli proteins are nearly identical ( Fig. 2a ), the protein–DNA contacts are also very similar. For example, there are five residues in both proteins that specifically recognize DNA base pairs (R35 in α2; R45 and T46 in α3; and H65 and G66 in the tip of the wing; Fig. 4b,c and Supplementary Fig. 3 ). There are also similarities in a number of nonspecific interactions with the DNA sugar–phosphate backbone, including A9, E34, T44, T47, R49 and T69 ( Fig. 4b,c and Supplementary Fig. 3 ). All contacts are symmetrical, except for T44, H65 and G66 (which have both symmetrical and non-symmetrical contacts) and K67 (which only has a non-symmetrical contact; Fig. 4b ). 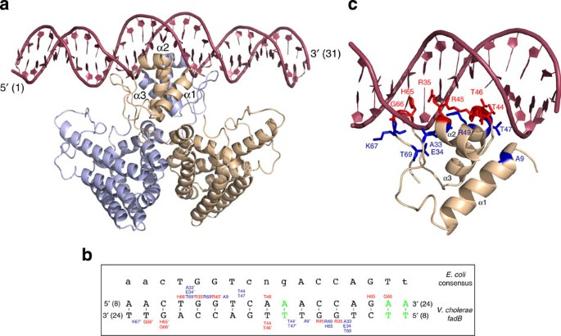Figure 4: Structure of theVcFadR–DNA complex. (a) TheVcFadR dimer bound to DNA. One monomer is slate blue and the other is wheat. (b) Schematic overview of theVcFadR–DNA contacts. Residues that form specific contacts with the DNA are red and those that form nonspecific interactions with the DNA sugar–phosphate are dark blue. The base pairs in theV. cholerae fadBrecognition sequence that are different from theE. coliconsensus sequence44are green. Within the consensus sequence, upper and lowercase letters represent nucleotides found more and less frequently, respectively. Residues from chain B are distinguished by a prime following the amino-acid number. (c) View showing a close up of theVcFadR–DNA interface within one monomer. Colours are the same as inb. Figure 4: Structure of the Vc FadR–DNA complex. ( a ) The Vc FadR dimer bound to DNA. One monomer is slate blue and the other is wheat. ( b ) Schematic overview of the Vc FadR–DNA contacts. Residues that form specific contacts with the DNA are red and those that form nonspecific interactions with the DNA sugar–phosphate are dark blue. The base pairs in the V. cholerae fadB recognition sequence that are different from the E. coli consensus sequence [44] are green. Within the consensus sequence, upper and lowercase letters represent nucleotides found more and less frequently, respectively. Residues from chain B are distinguished by a prime following the amino-acid number. ( c ) View showing a close up of the Vc FadR–DNA interface within one monomer. Colours are the same as in b . Full size image Superposition of the structures of the dimeric Vc FadR–DNA complex and the apo- Vc FadR dimer ( Fig. 5a ) shows that the DNA-binding domain and the insertion region are altered upon DNA binding. Within the DNA-binding domain, the distance between the two DNA recognition helices (α3) narrows from 17 Å in the apo- Vc FadR structure to 15 Å in the Vc FadR–DNA complex such that it is better able to interact with the DNA ( Fig. 5a ). In addition, the tip of the wing in each wHTH DNA-binding domain is shifted by 5 Å, forming interactions with DNA ( Fig. 5a ). 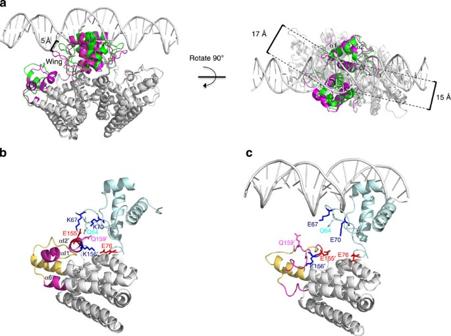Figure 5: Conformational changes inVcFadR upon DNA binding. (a) Superposition of theVcFadR–DNA complex and apo-VcFadR shown in two orientations (along and perpendicular to the pseudo twofold axis). The two primary regions that are altered upon DNA binding are shown in colour (green,VcFadR–DNA complex; magenta, apo-VcFadR) and the rest of the protein is white. The tip of the wing (H65) in each DNA wHTH-binding domain is shifted by up to 5 Å between the two structures and the distance between the two DNA recognition helices (R45 at the beginning of helix α3) is wider in apo-VcFadR structure (17 Å) compared with that in theVcFadR–DNA complex (15 Å). (b) Detailed view of the interaction between the insertion region and the wing of wHTH in the absence of the DNA. The N-terminal DNA-binding domain is pale cyan. The region that undergoes a helix-to-loop transition upon DNA binding (helices αI1, αI2 and the C-terminal end of α6 in apo-VcFadR) is magenta and the rest of the 40-residue insertion region is yellow. Residues that are positively charged are blue and those that are negatively charged are red. Helices and residues from chain B are distinguished by a prime. (c) Same view as inbbut in the presence of DNA. The colours are the same as inb. Figure 5: Conformational changes in Vc FadR upon DNA binding. ( a ) Superposition of the Vc FadR–DNA complex and apo- Vc FadR shown in two orientations (along and perpendicular to the pseudo twofold axis). The two primary regions that are altered upon DNA binding are shown in colour (green, Vc FadR–DNA complex; magenta, apo- Vc FadR) and the rest of the protein is white. The tip of the wing (H65) in each DNA wHTH-binding domain is shifted by up to 5 Å between the two structures and the distance between the two DNA recognition helices (R45 at the beginning of helix α3) is wider in apo- Vc FadR structure (17 Å) compared with that in the Vc FadR–DNA complex (15 Å). ( b ) Detailed view of the interaction between the insertion region and the wing of wHTH in the absence of the DNA. The N-terminal DNA-binding domain is pale cyan. The region that undergoes a helix-to-loop transition upon DNA binding (helices αI1, αI2 and the C-terminal end of α6 in apo- Vc FadR) is magenta and the rest of the 40-residue insertion region is yellow. Residues that are positively charged are blue and those that are negatively charged are red. Helices and residues from chain B are distinguished by a prime. ( c ) Same view as in b but in the presence of DNA. The colours are the same as in b . Full size image Although the insertion region (αI1, αI2 and several connecting loops) does not directly contact DNA ( Fig. 5a ), it undergoes a conformational change upon DNA binding. In the absence of DNA, the wing of the wHTH of chain A interacts with αI2 from the insertion region of chain B ( Fig. 5b ) via hydrogen bonds between the side chains of Q64 and K67 and the carbonyl oxygen of Q159′ (residues from chain B are distinguished by a prime) and two salt bridges (K70-E155′ and E76-K156′), suggesting the insertion stabilizes the wing. These interactions are also symmetric, although the distances are slightly longer between the insertion of chain A and the wing of chain B. In the presence of DNA ( Fig. 5c ), the wing of the wHTH moves away from the insertion to interact with DNA and helices αI1, αI2 and the C-terminal end of α6 undergo a helix-to-loop transition. This conformational change in the insertion region when Vc FadR is bound to DNA may be due to the loss of interactions with the wing. Structure of Vc FadR with ligand and comparison with Ec FadR In order to visualize the effects of ligand binding on Vc FadR, the structure was determined in the presence of the high binding affinity ligand, oleoyl-CoA [19] (18:1) ( Fig. 6a,b and Table 1 ). Interestingly, in contrast to Ec FadR, which binds one molecule of ligand (myristoyl-CoA (14:0) (PDB 1H9G) [17] ) per monomer ( Fig. 6c ), Vc FadR binds two ligand molecules, with one (coloured pink in Fig. 6a ) located in the site corresponding to the Ec FadR ligand-binding site (designated site no. 1) and the other (coloured yellow in Fig. 6a ) in a binding site derived in part from the 40-residue insertion region (designated site no. 2) that is structurally distinct from site no. 1 (electron density is shown in Supplementary Fig. 4 ). Thus, the insertion in FadR from Vibrionaceae facilitates the binding of a second molecule of ligand into each monomer; this has not been observed in any FadR structure that has been solved to date. 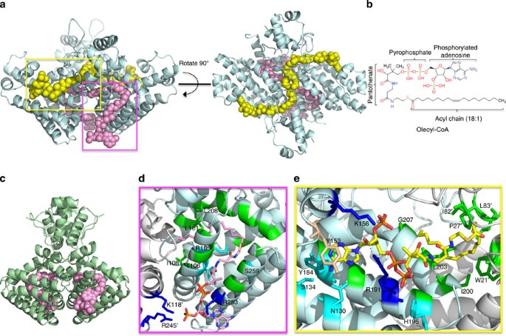Figure 6: Structures ofVcFadR andEcFadR with ligand. (a) TheVcFadR-oleoyl-CoA complex in two orientations. The ligand in the site corresponding toEcFadR (seec) is shown in pink spheres, whereas the ligand in the site that involves the insertion is in yellow spheres. (b) The chemical structure of oleoyl-CoA. (c) Structure ofEcFadR bound to myristoyl-CoA (PDB 1H9G)17. (d,e) Regions boxed inahighlighting critical residues interacting with the ligand in the pocket ofVcFadR corresponding to that ofE. coli(d, site no. 1, monomer A) and in the pocket derived from the insertion (e, site no. 2, monomer A). Positively charged residues that interact with ligand phosphates are in blue. Residues forming hydrogen bonds are cyan, and those forming hydrophobic interactions are in green. Y153, which forms π-stacking with adenosine of the ligand, is wheat. Residues from chain B are distinguished by a prime following the amino-acid number. The ligand is shown as sticks ind,e. The carbon atoms are coloured pink indand yellow ine. Other atoms of the ligand are coloured as follows: nitrogen, blue; oxygen, red; sulfur, dark yellow; phosphorous, orange. Figure 6: Structures of Vc FadR and Ec FadR with ligand. ( a ) The Vc FadR-oleoyl-CoA complex in two orientations. The ligand in the site corresponding to Ec FadR (see c ) is shown in pink spheres, whereas the ligand in the site that involves the insertion is in yellow spheres. ( b ) The chemical structure of oleoyl-CoA. ( c ) Structure of Ec FadR bound to myristoyl-CoA (PDB 1H9G) [17] . ( d , e ) Regions boxed in a highlighting critical residues interacting with the ligand in the pocket of Vc FadR corresponding to that of E. coli ( d , site no. 1, monomer A) and in the pocket derived from the insertion ( e , site no. 2, monomer A). Positively charged residues that interact with ligand phosphates are in blue. Residues forming hydrogen bonds are cyan, and those forming hydrophobic interactions are in green. Y153, which forms π-stacking with adenosine of the ligand, is wheat. Residues from chain B are distinguished by a prime following the amino-acid number. The ligand is shown as sticks in d , e . The carbon atoms are coloured pink in d and yellow in e . Other atoms of the ligand are coloured as follows: nitrogen, blue; oxygen, red; sulfur, dark yellow; phosphorous, orange. Full size image For the ligand bound to site no. 1 in monomer A, salt bridges are formed between ligand phosphates and residues R253, K118′ and R245′ ( Fig. 6d and Supplementary Fig. 5a ). In monomer B, the phosphorylated adenosine head group of the site no. 1 ligand has a different and more disordered conformation than that in monomer A ( Supplementary Fig. 6 ), and electron density can be observed for multiple positions of the head group. The arrangements of salt bridges in Vc FadR differ significantly from the Ec FadR-myristoyl-CoA structure (1H9G) [17] where only one salt bridge forms between the ligand phosphate and Ec FadR R213 (corresponding to Vc FadR R253). In Vc FadR, additional hydrogen bonds are formed between carbonyl oxygens in the pantothenic acid moiety and the polar side chains T106 and S259 ( Fig. 6d and Supplementary Fig. 5a ), homologous to hydrogen bonds involving Ec FadR T106 and S219). Finally, as in the Ec FadR-myristoyl-CoA structure (1H9G) [17] , the C18 acyl chain adopts a bent conformation and terminates in a hydrophobic pocket formed by residues L101, I108 and L208 from helices α5 and α8 ( Fig. 6d and Supplementary Fig. 5a ). The FadR ligand pocket thus can clearly accommodate ligands of different lengths, as the longer acyl chain in Vc FadR structure extends ~4 Å farther into the pocket compared with the C14 acyl chain of myristoyl-CoA in Ec FadR (1H9G) [17] . It is unclear from the structure if the unsaturated bond between C9 and C10 of oleoyl-CoA plays an important role in binding; however, comparison of the Vc FadR and Ec FadR pockets in this region does show one change that might be significant; M168 in Ec FadR is replaced by L208 in Vc FadR, which is positioned relatively further away from the ligand, perhaps to accommodate the kink in the fatty acyl chain introduced by the double bond ( Supplementary Fig. 7 ) For ligand-binding site no. 2, residues involved in specific interactions with the ligand are shown in Fig. 6e and Supplementary Fig. 5b . Both K156 from αI2 and R191 from α7 form salt bridges with ligand phosphate groups, and Y153 from αI2 forms a π-stacking interaction with the adenine ring. N130, S134 and Y184 form hydrogen bonds with the adenine ring ( Fig. 6e ). The C18 acyl chain is buried in a pocket surrounded by hydrophobic residues and the tails of the acyl chains from each monomer pack closely together ( Fig. 6a , right centre). The dominantly hydrophobic pocket is mainly formed by residues from helix α8 and the loop region connecting the DNA-binding and the ligand-binding domains (for example, I82′, L83′, I200, L203, G207; Fig. 6e and Supplementary Fig. 5b ). In addition, upon ligand-binding, residues in the DNA-binding domain (for example, W21′ and P27′) move closer to the C-terminal domain and interact with the ligand (see following section). Interestingly, the bent helix α8 (residues 199–221, notably G207) forms part of both binding sites no. 1 and no. 2. The above-mentioned residues that are interacting with ligand in binding site no. 2 are highly conserved among the other FadR proteins with the insertion ( Fig. 2b and Supplementary Fig. 1 ), suggesting that they will also bind the second ligand. To determine the thermodynamic parameters for binding of the oleoyl-CoA ligand to Vc FadR, isothermal titration calorimetry (ITC) was used to measure the dissociation constant ( K d ), enthalpy (Δ H ) and the stoichiometry of binding ( n ). Typical ITC profiles of the binding of oleoyl-CoA to Vc FadR are shown in Supplementary Fig. 8 . Consistent with the crystal structure, the stoichiometry of binding indicates that every monomer of Vc FadR protein binds two molecules of oleoyl-CoA. The biphasic nature of the isotherm indicates the presence of nonequivalent binding sites with different affinities for oleoyl-CoA (6 and 88 nM). Although it is not possible to determine which binding site has the higher affinity from the ITC data, computed scoring functions obtained from X-SCORE [24] and DSX [25] predict the higher-affinity binding pocket to be site no. 1. Comparison of effector-mediated conformational changes Having defined the structures of V. cholerae apo-FadR, FadR-DNA and FadR-oleoyl-CoA ligand complexes, a comparison can now be made between the effects of ligand binding on Vc FadR and Ec FadR. In Vc FadR, the linker helix α4, which is observed in the Vc FadR–DNA and apo- Vc FadR structures ( Fig. 7a,b and Supplementary Fig. 9 ), unwinds upon ligand binding to site no. 2 to avoid potential clashes with the ligand ( Supplementary Fig. 2c ). This transition also appears to destabilize the extensive hydrophobic contacts of α4 with the adjacent DNA-binding and ligand-binding domains ( Supplementary Fig. 9c ), enabling the DNA-binding domain to become uncoupled from the ligand-binding domain. 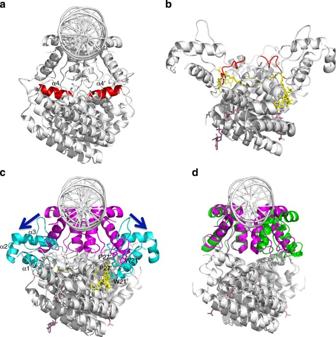Figure 7: Comparison of effector-mediated conformational changes betweenV. choleraeandE. coli. (a) TheVcFadR–DNA complex. The linker helix α4 is red and changes to a loop in theVcFadR–ligand complex (b). α4 from chain B is distinguished by a prime. (c) Superposition of the structures of theVcFadR–DNA complex andVcFadR–ligand complex. The DNA-binding domain is in magenta (VcFadR–DNA complex) or cyan (VcFadR–ligand complex) and the rest of the protein is white. The arrows show that, upon ligand binding, the DNA-binding domain is widened to almost 180°. Residues from chain B are distinguished by a prime following the amino-acid number. (d) Superposition of the structures ofEcFadR–DNA complex (PDB 1H9T)17andEcFadR–ligand complex (PDB 1H9G)17. The DNA-binding domain is magenta (EcFadR–DNA complex) or green (EcFadR–ligand complex) and the rest of the protein is white. Figure 7: Comparison of effector-mediated conformational changes between V. cholerae and E. coli . ( a ) The Vc FadR–DNA complex. The linker helix α4 is red and changes to a loop in the Vc FadR–ligand complex ( b ). α4 from chain B is distinguished by a prime. ( c ) Superposition of the structures of the Vc FadR–DNA complex and Vc FadR–ligand complex. The DNA-binding domain is in magenta ( Vc FadR–DNA complex) or cyan ( Vc FadR–ligand complex) and the rest of the protein is white. The arrows show that, upon ligand binding, the DNA-binding domain is widened to almost 180°. Residues from chain B are distinguished by a prime following the amino-acid number. ( d ) Superposition of the structures of Ec FadR–DNA complex (PDB 1H9T) [17] and Ec FadR–ligand complex (PDB 1H9G) [17] . The DNA-binding domain is magenta ( Ec FadR–DNA complex) or green ( Ec FadR–ligand complex) and the rest of the protein is white. Full size image Comparison of the Vc FadR-oleoyl-CoA and Vc FadR–DNA complexes shows that ligand binding induces the DNA-binding domain to move as a rigid body towards the C-terminal domain ( Fig. 7c ). This allows residues W21′ and P27′ from the DNA-binding domain to interact with the ligand ( Figs 6e and 7c ); in turn, this could stabilize the DNA-binding domain in this conformation. This movement leads to a large change in the distance between the two recognition helices (α3), from 15 Å in the Vc FadR–DNA complex (17 Å in the apo- Vc FadR structure) to 65 Å in the Vc FadR-oleoyl-CoA complex ( Fig. 7c and Supplementary Fig. 10a ). On the basis of these conformational changes, we propose that binding of the second ligand to Vc FadR induces a dramatic separation of the two recognition helices, strongly inhibiting the ability of Vc FadR to interact with DNA. In contrast to Vc FadR, ligand binding to Ec FadR does not alter the conformation of linker helix α4 as significantly. Instead of the unwinding of α4 described above, ligand binding to Ec FadR pushes α4 towards the N-terminal DNA-binding domain, where it forms additional contacts with helix α1. The resulting tilt in α1 moves the DNA-binding domain ~13° away from the DNA [17] . This results in smaller separation of the two recognition helices of Ec FadR than observed in Vc FadR, from 15 Å in the Ec FadR–DNA complex (PDB 1H9T; 15 Å in the apo- Ec FadR structure, PDB 1E2X) [16] , [17] to 23 Å in the Ec FadR-myristoyl-CoA structure (PDB 1H9G) [17] ( Fig. 7d and Supplementary Fig. 10b ). FadR is the master regulator of FA metabolism in bacteria and coordinately controls the pathways of FA degradation and UFA biosynthesis. In V. cholerae , FadR also regulates these processes, but the protein is different from other GntR family homologues in that it has a 40-residue insertion in its C-terminal domain. In all of the structures of FadR that have been solved to date, each monomer binds only one molecule of the acyl-CoA ligand. Although the overall structure of Vc FadR and the manner in which it binds to DNA described here is similar to Ec FadR, the insertion in the V. cholerae protein elongates the acyl-CoA-binding domain and accommodates a second ligand of oleoyl-CoA. One of these sites (site no. 1) is structurally similar to the ligand-binding site in Ec FadR, whereas the other (site no. 2) is comprised of residues from the insertion as well as from the N- and C-terminal domains of the protein. Although the two sites share some structural features, such as the involvement of residues within α8, Vc FadR appears to have evolved a new way to bind an additional molecule of the same ligand. We are aware of only two other transcription factors that have been shown to bind more than one molecule of the same ligand in distinct sites within a monomer. The E. coli catabolite gene activator protein was crystallized in the presence of DNA with two molecules of cAMP bound to each monomer (PDB 2CGP); however it is not clear whether binding of the second ligand is biologically relevant [26] . BenM, a LysR family transcription factor, was also crystallized with one molecule of benzoate bound at a primary site and another molecule of benzoate (PDB 2F78) bound at a secondary binding site within the same monomer; however, a different ligand, muconate, is also capable of binding at the primary site [27] . In the presence of both effectors, a unique conformation capable of high-level transcriptional activation is achieved [27] . The two ligand-binding sites in Vc FadR appear to have significantly different affinities for oleoyl-CoA. Site no. 1, the site structurally similar to Ec FadR, is predicted to be the higher-affinity site and appears to bind ligand with a higher affinity (6 nM) than the E. coli protein, determined for oleoyl-CoA to be 70 nM. In contrast, site no. 2, derived from the insertion, is predicted to be the lower-affinity site and binds ligand with a reduced affinity (88 nM) compared with the E. coli protein. Both site nos 1 and 2 of Vc FadR bind ligand with a higher affinity compared with Salmonella enterica (143 nM), Pasteurella multocida (2,231 nM) and Haemophilus influenzae protein (2,636 nM) [19] . Analysis of Vc FadR-binding site no. 1 shows a greater number of salt bridges are formed with ligand phosphates than for Ec FadR, and these additional interactions could be responsible for the increased affinity for ligand at this site. It is also possible that the presence of the insertion in Vc FadR alters the dynamics of the entire protein so as to increase the affinity for ligand at site no. 1 (ref. 28 ). For example, in addition to providing a second binding site for the ligand, the insertion also appears to stabilize the wing of the wHTH-binding domain in the absence of DNA. This interaction could change the protein such that its affinity for ligand increases. It has previously been shown that addition of oleate to V. cholerae FadR allows for nearly complete derepression of genes involved in FA utilization, suggesting that in the presence of ligand, Vc FadR decreases its affinity for DNA to a greater extent than other regulators [19] . These findings are consistent with our observation that the V. cholerae protein undergoes dramatic conformational changes upon ligand binding that would more fully disrupt DNA binding than the ligand-induced movements in Ec FadR and suggest that the binding of ligand to site no. 2 is physiologically relevant. In Vc FadR, ligand binding to site no. 2 induces a helix-to-loop transition in α4 that enables the DNA-binding domain to swing towards the C-terminal domain, forming stabilizing interactions with the site no. 2 ligand. We propose that this conformational change allows for a more complete release of the protein from the DNA, leading to fuller expression of the FA utilization genes. In addition, the presence of two binding sites with different affinities likely gives Vc FadR a broader response range to different concentrations of ligand than Ec FadR. For example, the model predicts that, at very low concentrations, Vc FadR binds only one ligand per monomer (likely at site no. 1) causing Vc FadR to have a reduced affinity for DNA, similar to that of Ec FadR. At higher concentrations of the ligand, Vc FadR binds two ligands per monomer (at both site nos 1 and 2), further reducing the affinity of the protein for DNA in comparison with Ec FadR. Unlike other enteric bacteria such as E. coli that colonize the digestive tract, Vibrionaceae are frequently found in aquatic environments where they acquire FAs from the sediment [29] , [30] . The need for Vibrionaceae to have a more efficient mechanism for utilizing FAs in this environment may have selected for an additional ligand-binding site in FadR that allows the protein to function as a more dynamic regulatory switch. Expression and purification of FadR V. cholerae FadR was purified using the IMPACT-CN fusion protein system (New England Biolabs). The full-length fadR gene was PCR-amplified from V. cholerae C6706 str2 using primers FadR5 and FadR6 ( Supplementary Table 1 ). The resulting fragment was inserted into pTXB1 (New England Biolabs) to produce the FadR-intein/CBD (chitin-binding domain) fusion construct pWEL225. FadR was expressed in BL21 (DE3) by autoinduction [31] in ZYM-5052 media. Cells were harvested by centrifugation, resuspended in column buffer (20 mM HEPES pH 7.8, 1 mM EDTA and 500 mM NaCl), lysed by sonication, clarified by centrifugation and filtered through a 0.45-μm filter. Chitin beads (New England Biolabs) were equilibrated with cold column buffer, mixed with the clarified supernatant and incubated at 4 °C with gentle rocking. The chitin bead slurry was then loaded on a gravity flow column, washed with 50 column volumes of high-salt wash buffer (20 mM HEPES pH 7.8, 1 mM EDTA and 1 M NaCl) and equilibrated with five column volumes of cleavage buffer (20 mM HEPES pH 7.8, 1 mM EDTA and 50 mM NaCl). The intein with the CBD was cleaved from FadR using cleavage buffer with 100 mM β-mercaptoethanol and left at 16 °C for 16 h. Eluant from the chitin column in cleavage buffer was then loaded on a new chitin column and followed by a HiTrap Sepharose prepacked (Q) fast flow (FF) strong anionic exchange column (GE) using a NaCl gradient. This separates the FadR-intein/CBD fusion protein and the intein tag that coeluted with the native FadR. The fractions containing FadR were identified by SDS–polyacrylamide gel electrophoresis and pooled. The pooled fractions were concentrated with an Amicon Ultra Centrifugal filter unit (Millipore) and applied to a Superdex 75 Prep Grade column (GE) equilibrated in crystallization buffer (20 mM HEPES pH 7.8, 1 mM EDTA and 100 mM NaCl). FadR eluted as a single peak at a position consistent with a dimer and was essentially pure as judged by SDS–polyacrylamide gel electrophoresis. To prepare the Vc FadR–DNA complex for crystallization, the oligonucleotides WS1 and WS2 ( Supplementary Table 1 ) were dissolved in low-salt buffer (100 mM NaCl and 10 mM NaOH) and purified using MonoBeads prepacked Mono Q strong anionic exchange column (GE) with a NaCl gradient in 10 mM NaOH. The fractions containing pure oligonucleotides were pooled and concentrated as described above and the buffer was exchanged into crystallization buffer by a desalting column (GE). The purified oligonucleotides were annealed, concentrated and applied to a Superdex 75 Prep Grade column (GE) equilibrated in crystallization buffer to eliminate unannealed oligonucleotides. The purified double-stranded DNA was mixed with purified Vc FadR at a protein/DNA ratio of 1:1.5. The Vc FadR–DNA complexes were concentrated as described above and applied to a Superdex 200 Prep Grade column (GE) equilibrated in crystallization buffer. The fractions containing the Vc FadR–DNA complexes were collected and concentrated as described above. Crystallization Crystals of apo- Vc FadR were obtained using the sitting drop procedure by mixing equal volumes of the protein solution at 6 mg ml −1 with a reservoir solution containing 0.2 M sodium chloride, 0.1 M MES pH 6.5, 10% (w/v) PEG 4000. Crystals typically grew within 1 week. Vc FadR crystals were cryoprotected in a 30% v/v solution of glycerol/mother liquor and flash-frozen in liquid nitrogen for X-ray data collection. Crystals of the Vc FadR–DNA complex were also obtained by the sitting drop method by mixing equal volumes of 8 mg ml −1 complex solution with a reservoir containing 0.2 M lithium sulfate, 0.1 M Tris pH 8.5 and 1.26 M ammonium sulfate. Crystals grew in 2 weeks. Vc FadR–DNA complex crystals were cryoprotected in a 30% v/v solution of glycerol/mother liquor and flash-frozen in liquid nitrogen for X-ray data collection. Crystals of the Vc FadR-oleoyl-CoA complex, also obtained by the sitting drop method, were produced by mixing equal volumes of the Vc FadR–ligand complex ( Vc FadR=4 mg ml −1 ; ligand (oleoyl coenzyme A lithium salt (Sigma))/ Vc FadR monomer molar ratio=3.6:1) solution with a reservoir containing 17% PEG 3350, 0.23 M magnesium formate. Crystals grew in about 1 week. Vc FadR-oleoyl-CoA complex crystals were cryoprotected in a 30% v/v solution of glycerol/mother liquor and flash-frozen in liquid nitrogen for X-ray data collection. Data collection and structure solution Crystals of apo- Vc FadR diffracted to 2.2 Å at NSLS beamline X6A at the Brookhaven National Laboratory. Crystals belonged to the tetragonal space group P4 1 with unit cell dimensions a =87.48 Å, b =87.48 Å, c =81.43 Å, α =90.0°, β =90.0°, γ =90.0°. The asymmetric unit contained one dimer of Vc FadR, giving a crystal volume per protein mass ( V M ) of 2.4 Å 3 Da −1 and a solvent content of 49.7%. Data were processed in XDS [32] and structure determination was carried out using AutoMR in Phenix [33] . Two copies of the E. coli FadR monomer divided into the N-terminal (residues 6–137) and C-terminal domain (residues 138–226) were used as search models for molecular replacement. The insertion region was built back manually in Coot [34] . Multiple rounds of refinement and rebuilding were carried out in Phenix.refine [35] and Coot [34] , respectively, using data to 2.2 Å. The resulting final structure has a R-work 17.44% of and R-free of 20.46% with good stereochemistry ( Table 1 ) and continuous density for the backbone from residue 2 to 279 out of 279 possible residues ( Fig. 3a ). Ramachandran statistics show that 97% and 2.82% of the residues are in the preferred and allowed regions, respectively. In MOLPROBITY [36] validation results, this structure was assigned a MOLPROBITY score of 1.44, which is the 99th percentile among structures of comparable resolution. Diffraction data for the Vc FadR–DNA complex were collected to 3.2 Å at NSLS beamline X6A at the Brookhaven National Laboratory. Crystals belonged to the triclinic space group P1 with unit cell dimensions a =84.6 Å, b =94.7 Å, c =101.7 Å, α =89.8°, β =114.6°, γ =116.5°. The asymmetric unit contained two molecules of the Vc FadR–DNA complex, giving a crystal volume per protein mass ( V M ) of 3.9 Å 3 Da −1 and a solvent content of 71.0%. Data were processed in XDS [32] and structure determination was carried out using AutoMR in Phenix [33] . Four copies of the V. cholerae FadR monomer without the insertion region and two copies of DNA from E. coli FadR–DNA complex were used as search models for molecular replacement. The resulting maps showed density for the insertion region and density for additional DNA duplex. The insertion region was built back manually in Coot [34] ; the DNA duplex was mutated to the V. cholerae FadR DNA sequence and additional bases were built back manually in Coot [34] . Multiple rounds of refinement and rebuilding were carried out in Phenix.refine [35] and Coot [34] , respectively, using data to 3.2 Å. The resulting final structure has a R-work of 21.76% and R-free of 25.23%, with good stereochemistry ( Table 1 ) and continuous density that included all atoms in DNA and residues from residue 6 to 277 out of 279 possible residues ( Fig. 4a ). Ramachandran statistics show that 91% and 7.6% of the residues are in the preferred and allowed regions, respectively. In MOLPROBITY [36] validation results, this structure was assigned a MOLPROBITY score of 2.55, which is the 96th percentile among structures of comparable resolution. Diffraction data for Vc FadR with ligand were collected to 2.8 Å at NSLS beamline X6A at the Brookhaven National Laboratory. Crystals belonged to the orthorhombic space group P2 1 2 1 2 1 with unit cell dimensions a =116.92 Å, b =88.69 Å, c =62.86 Å, α =90°, β =90°, γ =90°. The asymmetric unit contained one dimer of the Vc FadR-oleoyl-CoA complex, giving a crystal volume per protein mass ( V M ) of 2.4 Å 3 Da −1 and a solvent content of 48.4%. Data were processed in XDS [32] and structure determination was carried out using AutoMR in Phenix [33] . Initial molecular replacement with V. cholerae apo-FadR as a search model, was unsuccessful, suggesting that significant structural rearrangement might have occurred upon binding of oleoyl-CoA. Subsequent molecular replacement with only the C-terminal acyl-CoA-binding domain gave a single solution. Refinement in Phenix [35] resulted in maps in which the ligands and the N-terminal DNA-binding domain could be positioned manually in Coot [34] . Multiple rounds of refinement and rebuilding were carried out in Phenix.refine [35] and Coot [34] , respectively, using data to 2.8 Å. The resulting final structure has a R-work of 25.57% and R-free of 30.35%, with good stereochemistry ( Table 1 ) and continuous density that included all atoms in the ligand and residues from residue 8 to 266 out of 279 possible residues ( Fig. 5b ). Ramachandran statistics show that 87% and 6.8% of the residues are in the preferred and allowed regions, respectively. In MOLPROBITY [36] validation results, this structure was assigned a MOLPROBITY score of 3.15, which is the 53rd percentile among structures of comparable resolution. Construction of V. cholerae strains and mutations The fabA-lacZ fusion was constructed by amplifying a DNA fragment from C6706 str2 using primers FabA1 and FabA3 ( Supplementary Table 1 ). The fragment, together with a promoterless lacZ fragment from pVC200 (ref. 37 ), were inserted into pKAS180 (ref. 38 ) generating pWEL234. Plasmid pWEL234 was used for allelic exchange [38] into the lacZ locus of V. cholerae strain KSK262 (ref. 39 ) generating WL1005. Plasmid pWEL236 was constructed by amplifying a DNA fragment from C6706 str2 using primers Chr1 and Chr2 and a DNA fragment from pVC200 (ref. 37 ) using primers LacNot and LacBgl. The resulting fragments were inserted into pKAS154 (ref. 40 ). The fadE , fadBA , fadH and fabB-lacZ fusions were constructed by amplifying DNA fragments from C6706 str2 using primers FadE1 and FadE3, FadB1 and FadB4, FadH1 and FadH3, and FabB3 and FabB4. The resulting fragments were inserted into pWEL236, generating plasmids pWEL239, pWEL240, pWEL242 and pGKK469, respectively. The fusions in the resulting plasmids were introduced into the lacZ locus of KSK262 by allelic exchange generating strains WL1027, WL1031, WL1040 and GK1609. The Δ fadR mutation was constructed by amplifying two DNA fragments from C6706 str2 using primers FadR1 with FadR2 and FadR3 with FadR4. The fragments were inserted into pKAS154 (ref. 40 ), generating plasmid pGKK367, and the deletion was introduced into the chromosome of V. cholerae by allelic exchange. β-Galactosidase assays β-Galactosidase assays [41] were carried out by growing cultures in Tryptone medium with aeration for 5 h at 37 °C. How to cite this article : Shi, W. et al . The 40-residue insertion in Vibrio cholerae FadR facilitates binding of an additional fatty acyl-CoA ligand. Nat. Commun. 6:6032 doi: 10.1038/ncomms7032 (2015). Accession codes: Atomic coordinates and structure factor files have been deposited in the Protein Data Bank (ID codes: apo- Vc FadR, 4P96 ; Vc FadR–DNA complex, 4P9U ; Vc FadR–ligand complex, 4PDK ).